Spatial modulation of light transmission through a single microcavity by coupling of photosynthetic complex excitations to surface plasmons Molecule–plasmon interactions have been shown to have a definite role in light propagation through optical microcavities due to strong coupling between molecular excitations and surface plasmons. This coupling can lead to macroscopic extended coherent states exhibiting increment in temporal and spatial coherency and a large Rabi splitting. Here, we demonstrate spatial modulation of light transmission through a single microcavity patterned on a free-standing Au film, strongly coupled to one of the most efficient energy transfer photosynthetic proteins in nature, photosystem I. Here we observe a clear correlation between the appearance of spatial modulation of light and molecular photon absorption, accompanied by a 13-fold enhancement in light transmission and the emergence of a distinct electromagnetic standing wave pattern in the cavity. This study provides the path for engineering various types of bio-photonic devices based on the vast diversity of biological molecules in nature. The interaction between molecules and surface plasmons (SP) in defined geometries can lead to new light–matter hybrid states, where light propagation is strongly influenced by molecular photon absorption [1] , [2] , [3] , [4] , [5] , [6] , [7] , [8] , [9] , [10] , [11] , [12] , [13] , [14] . This phenomenon has been observed in organic semiconductor optical microcavities [3] , [11] , [12] , [13] , sub-wavelength hole arrays [1] , [9] , [10] and molecules deposited on patterned surfaces [1] . The applications range from lasing [15] , LED’s [12] , control of chemical reactions [11] and light harvesting [2] , [16] , [17] . In this respect, it is intriguing to explore the opto-electronic properties of hybrid systems comprising molecules, which exhibit highly efficient, long-range exciton energy transfer. Of a special interest is the photosynthetic light harvesting complex, photosystem I (PS I) [18] , [19] , [20] , [21] , [22] . Photosynthetic complexes are evolutionary tuned to efficiently capture solar light. The initial steps of photosynthesis involve the absorption of photons by pigment molecules located in a protein antenna matrix, which is followed by rapid and highly efficient funnelling of exciton energy to power the reaction centres in these specialized biological light-to-chemical energy converters. There is compelling experimental evidence that long-lived electronic quantum coherence and entanglement play an important part in energy transfer processes in such systems, even at physiological temperatures [23] , [24] , [25] . Here, we report on the first successful attempt to integrate PS I proteins in a single microcavity and elucidate light transmission mechanism through the hybrid system. A spatial modulation of light transmission (SMOL) through a single microcavity patterned on a free-standing Au film, coupled to PS I is observed. A distinct correlation between this phenomenon and the PS I’s absorption is demonstrated and simulated. The effect is visualized as a standing wave pattern accompanied by a 13-fold enhancement in light transmission. Preparation of the hybrid system We experimentally study and simulate light transmission through a hybrid system composed of a microscopic cavity drilled in a free-standing 200-nm-thick Au metal film decorated with self-assembled single and multilayers of PS I, covalently bonded to the cavity walls (see Fig.1 and methods section) . The PS I used in this study, derived from cyanobacterial membrane, is a nanosize protein–chlorophyll complex, which integrates 96 chlorophyll and 22 carotenoid pigment molecules in a helical protein membrane complex. It harvests photons with a quantum efficiency of ∼ 1, and was found to be stable and photoactive when adsorbed in a dry environment [19] , [26] , [27] , [28] . Self-assembled mono and multilayers of PS I were fabricated by formation of a direct sulfide bond between unique cysteine mutants in PS I and the patterned Au surface (see Fig. 2a,b , Supplementary Fig. 1 and Methods section) [19] . The advantage of this technique compared with spin coating, in which the entire hole is covered with the thick organic layer, is that here the surface of the metal and the slit circumference are fully coated with only a thin (few tenths of nanometre) organized organic layer, leaving the majority of the slit void ( Fig. 2b ). 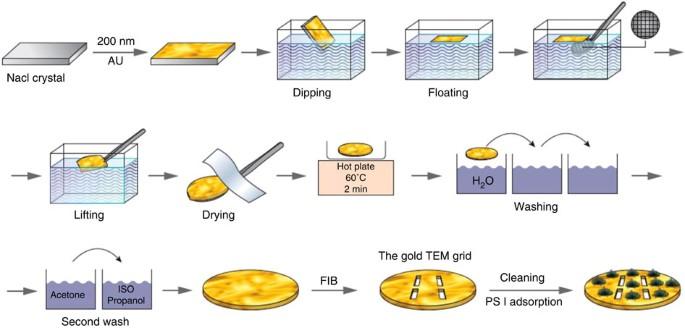Figure 1: Fabrication of the PS I - single microcavity hybrid system. Schematic illustration of the microcavity fabrication in a thin free-standing metal film and the PS I molecular film coating on the Au surface. Figure 1: Fabrication of the PS I - single microcavity hybrid system. Schematic illustration of the microcavity fabrication in a thin free-standing metal film and the PS I molecular film coating on the Au surface. 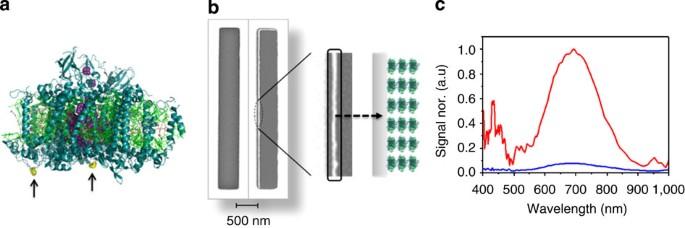Figure 2: Coupling of PS I to a free-standing Au microcavity. (a) PS I structure. The cysteine mutations used to bind the PS I to the metal surface are depicted in yellow space-filled sulfur atoms and indicated by arrows. (b) Left: SEM images of an uncoated 440 × 4,500 nm single slit (left) and a slit that is adsorbed with three PS I layers (right). Right: zoom of the coated slit corresponds to layer thickness of 33±4 nm (three layers) that is formed on the walls of the slit, leaving the majority of the slit vacant. (c) Normalized transmission of light through 440 × 4,500 nm single slit adsorbed with a multilayer composed of three PS I layers (red), in comparison with transmission through an uncoated slit (blue). Transmission of light (far-field) through the coated slit is enhanced by a factor of 13 in comparison with the slit not coated with molecules. Full size image Figure 2: Coupling of PS I to a free-standing Au microcavity. ( a ) PS I structure. The cysteine mutations used to bind the PS I to the metal surface are depicted in yellow space-filled sulfur atoms and indicated by arrows. ( b ) Left: SEM images of an uncoated 440 × 4,500 nm single slit (left) and a slit that is adsorbed with three PS I layers (right). Right: zoom of the coated slit corresponds to layer thickness of 33±4 nm (three layers) that is formed on the walls of the slit, leaving the majority of the slit vacant. ( c ) Normalized transmission of light through 440 × 4,500 nm single slit adsorbed with a multilayer composed of three PS I layers (red), in comparison with transmission through an uncoated slit (blue). Transmission of light (far-field) through the coated slit is enhanced by a factor of 13 in comparison with the slit not coated with molecules. Full size image Light transmission measurements Transmission spectra and images (recorded by a CCD (charge-coupled device) in the far-field region) of individual single slits (PS I-coated and uncoated) with various dimensions are shown in Fig. 2c and Fig. 3 (see also Supplementary Fig. 2 and Methods section). The spectral response exhibit a pronounced enhancement (13-fold) in light transmission through slits coated with three PS I layers ( Fig. 2b,c ) compared with uncoated slit. The resulting transmission images ( Fig. 3 ) indicate that light is transmitted in a spatially smooth and continuous manner in the case of the bare slit ( Fig. 3a ). Small deformation of light transmission is observed for cavities coated with a single PS I layer ( Fig. 3b ). Remarkably, when the surface of the slit is coated with three PS I layers, light emerges as circles dividing the slit into several distinct bright spots ( Fig. 3c–e ). These results are a clear indication that the observed SMOL phenomenon is due to the presence of the PS I layers. To exclude that SMOL solely originated from geometrical effects, we have investigated uncoated slits of various dimensions. In all the cases, no evidence for SMOL was found ( Supplementary Fig. 3 ). Polarization experiments revealed that SMOL is only weakly dependent on light polarization ( Supplementary Fig. 4 ). In addition, evidence has been found that the energy-dispersion spatial dependence within the slit is correlated with the molecular optical adsorption ( Supplementary Figs 5 and 6 ). Coupling the cavities to other molecular systems such as porphyrins, polypeptides and saturated monolayers of hydrocarbon did not yield SMOL. 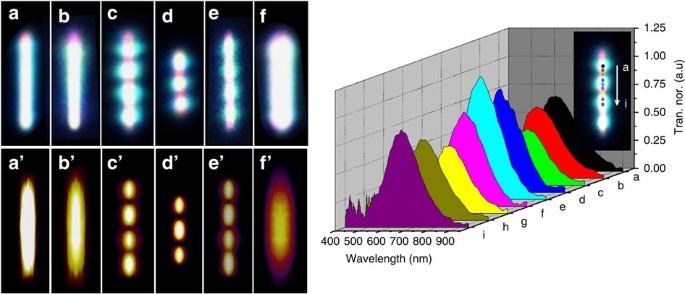Figure 3: Experiments and simulations of light transmission through single individual slits in the far-field region. Left: transmission of white light through coated and uncoated slits (a–f) and the corresponding 3D simulation (a'–f'); (a) an uncoated 440 × 4,500 nm slit, (b) 440 × 4,500 nm slit decorated with single PS I monolayer (1PSI), (c) 440 × 4,500 nm slit coated with three PS I layers (3PSI), (d) 440 × 3,000 nm (3PSI), (e) 220 × 4,500 nm (3PSI), (f) 900 × 4,500 nm (3PSI). Bright circles of light appear in slits coated with3PSIfor slits width <680 nm. (a'–f') Simulation of far-field transmitted light through the various slits. Right: spatial modulation of light transmission across the slit inFig. 2c. Inset: scan direction is from point a to i. Light transmission intensity is modulated across the slit with maximum intensities at the centre of the light circle and minimum at the nodes between two adjacent circles. Each spectrum was taken from an area cross-section of∼80 × 80 nm2of the CCD image. nor., normalized; Tran., transmission. Figure 3: Experiments and simulations of light transmission through single individual slits in the far-field region. Left: transmission of white light through coated and uncoated slits ( a – f ) and the corresponding 3D simulation (a'–f'); ( a ) an uncoated 440 × 4,500 nm slit, ( b ) 440 × 4,500 nm slit decorated with single PS I monolayer ( 1PSI ), ( c ) 440 × 4,500 nm slit coated with three PS I layers ( 3PSI ), ( d ) 440 × 3,000 nm ( 3PSI ), ( e ) 220 × 4,500 nm ( 3PSI ), ( f ) 900 × 4,500 nm ( 3PSI ). Bright circles of light appear in slits coated with 3PSI for slits width <680 nm. (a'–f') Simulation of far-field transmitted light through the various slits. Right: spatial modulation of light transmission across the slit in Fig. 2c . Inset: scan direction is from point a to i. Light transmission intensity is modulated across the slit with maximum intensities at the centre of the light circle and minimum at the nodes between two adjacent circles. Each spectrum was taken from an area cross-section of ∼ 80 × 80 nm 2 of the CCD image. nor., normalized; Tran., transmission. Full size image The appearance of this pronounced SMOL does not depend on the width of the slit up to 680 nm. However, at larger widths (900 nm slit, Fig. 3f ), the SMOL effect is lost, indicating that both molecular absorption and light geometric resonances play an important role in this phenomenon. A representative spectral response of the spatially resolved light transmission is shown in Fig. 3 —right. Light intensity across the slit longitudinal axis is modulated with minimum transmission at the nodes and maximum transmission in the centre of the circles. Simulations A corresponding simulation performed by a full three-dimensional (3D) numerical solution of Maxwell’s equations via finite element method (FEM) using adaptive mesh refinement process, reproduced the main spectral features observed. The simulation is in one-to-one correspondence with the experimental conditions and the sample parameters and compares between uncoated slits and slits coated with one or three PS I layers. The FEM was used to properly adapt the numerical computational accuracy to the spatially varied distribution of the simulated microstructures ( Fig. 3a'–f' and Supplementary Information ). Supplementary Fig. 7 shows the 3D electromagnetic model used to obtain the fields solution. In this model, the slit is illuminated from the bottom by optical sources at varied frequencies, with the entire aperture interacting with the light beam. The electric field corresponds to unpolarized radiation, and the wave vector K is perpendicular; corresponding to a normal incidence angle. A selectively dense meshing is assigned in the metallic and waveguide regions, with maximum cell size of 1 nm and 1,000,000 FEM tetrahedral cells as shown in Supplementary Fig. 8 , which displays the mesh for a converged solution. The macroscopic response of the molecular layer is modelled by its complex dielectric function; whose imaginary part governs light absorption while the real part is related to the energy stored in the medium. The PS I dielectric function, ɛ ( ω ), was calculated using: ɛ ( ω )= ɛ 1 ( ω )+ iɛ 2 ( ω ). The imaginary part of the dielectric function, ɛ 2 ( ω ), was extracted from an experimentally obtained frequency-dependent absorption coefficient [20] and ɛ 1 ( ω ), the real part was calculated using Kramers–Kronig relations analytically connecting the real and the imaginary parts of the dielectric function (Methods section and Supplementary Figs 9 and 10 ). Wavelength dependent SMOL Investigation of the SMOL with respect to the PS I absorption spectra ( Fig. 4 , right) is followed. 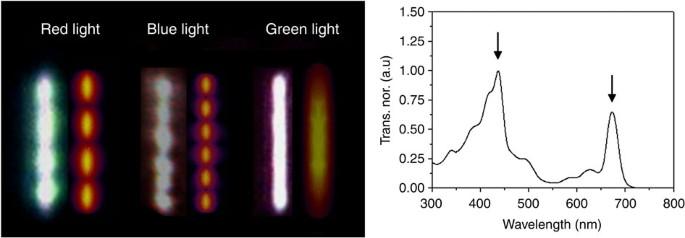Figure 4: Dependence of light transmission on PS I absorption bands. Left: the dependence of transmission on the wavelength of the transmitted light. Blue and red light are spatially modulated when transmitting through a 440 × 4,500 nm slit coated with3PSI, forming SMOL, while green light transmission shows negligible spatial modulation. Simulations are depicted on the right side of each slit. Right: excitation spectra of the PS I in solution. Two distinct absorption bands pointed by black arrows, in the blue (440 nm) and in the red (680 nm) are resolved. The spectra and simulation are both taken in the far-field region. nor., normalized; Trans., transmission. Figure 4 (left) shows transmission images taken under excitations in three main bands: blue (420–480 nm), green (510–550 nm) and red (600–800 nm). Notably, the transmission spectra significantly differ for each excitation band revealing four distinct circles of light under red band excitation, six for blue, whereas excitation by green light does not yield any SMOL effect. These results (supported by 3D simulations taken at the centre excitation frequency of each band, Fig. 4 , left) provides direct evidence that a strong SMOL takes place only at wavelengths in which the PS I absorbs light (red, blue and white) and does not occur under green excitation in which the PS I optical activity is low. Thus, the standing waves pattern observed can be directly related to molecular excitation of the PS I coupled to the plasmon cavity modes. Notice that the SMOL of the white light is similar to that of red light (in contrast to blue). This similarity is due to the fact that the intensity of the light source used is higher at longer wavelengths around the red region, and the Au plasmon response is weaker at shorter wavelengths (blue). Simulation of light transmission at selected wavelengths through an uncoated slit (depicted in Supplementary Fig. 11 ) reveals only a weak transmission pattern with negligible dependency on the excitation wavelength. Apparently, the PS I act as a nanophotonics filter, which selects the frequencies of the incoming photon to interact with the metallic cavity and enhances the plasmon excitation at the selected frequencies. An example of a possible application based on the SMOL effect, is a photon to digital converter, described at the Supplementary Information section ( Supplementary Fig. 12 ). Figure 4: Dependence of light transmission on PS I absorption bands. Left: the dependence of transmission on the wavelength of the transmitted light. Blue and red light are spatially modulated when transmitting through a 440 × 4,500 nm slit coated with 3PSI , forming SMOL, while green light transmission shows negligible spatial modulation. Simulations are depicted on the right side of each slit. Right: excitation spectra of the PS I in solution. Two distinct absorption bands pointed by black arrows, in the blue (440 nm) and in the red (680 nm) are resolved. The spectra and simulation are both taken in the far-field region. nor., normalized; Trans., transmission. Full size image The unique role of the PS I in SMOL formation can be attributed to two of the molecule’s distinct properties; the high absorption coefficient of its core pigments [21] and efficient exciton transfer. It is well documented that efficient long-range exciton transfer between the protein’s pigments is one of the most remarkable properties of the PS I antenna system [21] . This process may sustain efficient exciton transfer to the SP without considerable energy losses. Additional requirement for SMOL to take place is the existence of a dielectric coating comprised of several molecular layers. Thus, we predict the formation of SMOL in molecular systems fulfilling the above-indicated requirements. Potential candidates are J-aggregates [7] , bacteriorhodopsin, quantum dot hybrid systems [8] , photoactive proteins such as PS II and light harvesting complexes [23] , [24] , [25] arranged in an organized and oriented fashion of several layers thick. In summary, we have constructed and simulated a nano-sized solid-state biological hybrid system in which the active component is a PS I complex that functions as an antenna system, which captures light efficiently (at the excitation bands) and transfers it to the strongly coupled cavity SP. The incident photons are converted to surface plasmons, channel through the cavity and re-couple to radiating photons observed as SMOL and accompanied by a large enhancement in light transmission. The PS I act as a nanophotonic filter, which selects the frequencies of the photons to interact with the metallic cavity and excite the optical plasmons. Our simple imaging technique enables to visualize coupling between molecular excitations and SP and paves the way to further study and detection of fundamental microscopic properties of organic and biological molecules solid-state nano-hybrid systems. Fabrication of the hybrid system First a free-standing Au film on a TEM grid was formed ( Fig. 1 ). This was achieved by evaporating 200 nm Au on a NaCl crystal (Agar Scientific). The rate of evaporation was 0.7 A s −1 for the first 20 nm and then increased to 2 A s −1 . After evaporation, the crystal was cut into ∼ 3 mm 2 pieces and placed in a Petri dish of deionized water until the gold leaf was detached from the crystal and floated on the water surface. The gold leaf was then mounted on an Au TEM grid (SPI supply), dried with clean-room paper and placed for 2 min on a hot plate (60 °C) for further drying. The TEM grid was then washed in acetone and isopropanol and dried in air. In the second step, slits of different dimensions were drilled with a Raith ionLine focused ion beam, working with a beam of galium at 35 kV with a current of 40 pA. Adsorption of PS I monolayer was achieved by first cleaning the Au grid by Ar and O 2 (50%:50%) plasma. The grids were then washed in EtOH for 2 min, dried and placed in a concentrated solution of PS I for 2 h and washed in buffer and deionized water. Multilayers were fabricated by crosslinking of successive PS I layers. This technique insures that the PS I multilayer is covalently bound to the surface in an oriented fashion. Sample characterization Atomic force microscopy was used to evaluate the density and thickness of the PS I film formed on the Au surface. As indicated by AFM, the PS I forms dense mono and multilayers on the Au surface ( Supplementary Fig. 1 ). The granularity and height increase with the number of PS I layers adsorbed. Ellipsometry measurements indicated thicknesses of 10±2 nm and 36±4 nm for the PS I mono and multilayer, respectively. The imaging set-up The sample (Au leaf on a TEM grid) was placed on top of a 2-mm hole in a plastic microscope slide and attached to the sides of the hole ( Supplementary Fig. 2 ). The microscope slide was than located on the stage and centred at the beam. The light, of general polarization, that is, unpolarized light, was provided by a 100 W quartz halogen lamp at the base of the microscope (field diaphragm). The light enters the condenser, and after passing through the sample, it passes through a × 100-magnifying objective, which gives an image to the CCD. The CCD is capable of giving the spectral response at any given point of the image with a spatial resolution of 32 nm and wavelength spectral resolution full-width at half-maximum of 6 nm. The spectral response is given by dividing the transmission spectra of the light passing through the sample with a blank reference (same illumination condition with the absence of a sample). The CCD exposure is adjusted to the light intensity reaching the CCD (normalization of image light intensity). The change in this exposure condition is then taken into account when calculating the light intensity output from each slit. The light intensity entering the slit is the same in all the cavities. For testing the effect of light wavelength on transmission, colour filters were used. The filters were placed in the beam path before it enters the condenser. The filters used transmit light in the blue (420–480 nm), green (510–550 nm) and red (600–800 nm). Size-dependent transmission through uncoated slits Light transmission through slits of different lengths and width of 440 nm was studied and is depicted in Supplementary Fig. 3 . As can be seen through the images, there is no sign for SMOL effect in slits, which are uncoated with PS I. Polarization study Polarization experiments were performed on a 440 nm by 3 μm slit coated with 3PSI ( Supplementary Fig. 4 ).The results indicate that SMOL effect persists in both parallel and perpendicular polarizations. A reduction in the intensity of the light transmitted in per polarization is observed as expected, due to the smaller dimension of the slit width than its length. Dispersion-dependent light transmission The energetic profile of light-dependent spatial dispersion across the 440 × 3,000 nm slit ( Supplementary Fig. 5 corresponding to slit d in Fig. 3 ) indicates that the transmitted energy of light is spatially modulated across the slit. Apparently, the spectrum at the centre of the white circle is composed of two contributions; one which originates from the centre of the circle (636 nm), and a shoulder (710 nm) originating from the node. The energies of the two transmission peaks at 636 nm and 716 nm are distributed evenly on both sides of the excitation energy of the PS I (680 nm), with a separation of 230 meV. This energy distribution is supported by statistical measurements taken for 12 individual slits ( Supplementary Fig. 5 , right). It is important to note that while spatial dependent energy dispersion was observed across all the slits, as indicated in Supplementary Fig. 5 (right), local energy splitting in a narrow spectral region (10 4 nm 2 ) was only observed in the short slit (440 × 3,000 nm). The blue, brown and cyan curves of Supplementary Fig. 5 (left) each represent spectra taken at a local position, depicted by the dots in the inset. Each of these curves is composed of two spectral contributions. This is made evident by fitting a Lorentzian to the spectra ( Supplementary Fig. 6 ). As seen in the figure, each spectrum is composed of two spectra distributed (red curves) on both sides of the excitation energy of the PS I at 680 nm (black dotted line). The amplitude of the long wavelength energy Lorentzian, on the right side of the PS I excitation energy (at 680 nm) increases as the scan proceeds from the centre of the white circle towards the node. Comparing the 4.5-μm long slit to the shorter 3-μm slit ( Fig. 3c,d , respectively), we note that the transmission of light through the shorter slit has a more well-defined shape. The circles of light are brighter with clear separation (nodes). We suggest that the strong plasmon field in the shorter slit cause the initiation of a gap in the distribution of transmission energy at the PS I excitation energy. The result points to a correlation between the strength of the spatial modulation and the initiation of an energy gap and provides additional indication to the important role the PS I excitation play in light transmission through the coupled PS I single-slit hybrid system. Simulations The numerical results are obtained by using ANSYS HFSS V15 software package, the industry-standard simulation tool for 3D full-wave electromagnetic field simulation. HFSS solve Maxwell’s equations via the FEM using adaptive mesh refinement process for tailored accuracy requirements. HFSS was recently demonstrated in rigorous analysis and design of nanoplasmonic devices operating at optical frequencies [29] , [30] . The field’s solutions are calculated with the metallic (Au) plasmonic single slits being fully coated with PS I layers with parameterized thickness and material properties obtained from refs 20 , 31 , 32 . Supplementary Fig. 7 shows the 3D electromagnetic model used to obtain the fields solution. The device is illuminated from the bottom by optical sources at varied frequencies, with the entire aperture interacting with the light beam. The electric field is of general polarization, and the wave vector K is perpendicular; corresponding to normal incidence angle. A selectively dense meshing is assigned in the metallic and waveguiding regions, with maximum cell size of 1 nm and 1,000,000 FEM tetrahedral cells as shown in Supplementary Fig. 8a , which plots the mesh for converged solution. To provide maximum accuracy, the model is terminated as following: the interface with free space is bounded by perfectly matched layer absorbing boundary conditions, while the metallic and PS I termination are done via layered impedance absorbing boundary conditions. The minimum number of adaptive meshing iterations was set to 12, with convergence condition of 1% maximum energy variance between adjacent iterations. The adaptive mesh refinement ( Supplementary Fig. 8b ) shows the difference in energy between the stages of mesh refinement as a function of meshing iteration. It is observed that after five iterations of mesh refinement, the solution was converged and 1% energy difference between the successive iterations is achieved. Calculation of the dielectric function of PS I The dielectric function of the PS I can be described as: The imaginary part of the dielectric function was extracted from an experimentally obtained frequency-dependent absorption coefficient as observed in ref. 20 . The relation between absorption and the dielectric coefficient is as follows: where n is the average refraction index, c is the speed of light in free space, ω is the angular frequency and α abs is the absorption coefficient [31] . The real part of the dielectric coefficient is obtained using Kramers–Kronig relations: In the above equations, P denotes the Cauchy principal value. So realizing the first row of the above equation allowed translating the experimental approximations for ɛ 2 of ref. 20 into ɛ 1 . The macroscopic optical properties of Au were obtained from ref. 32 . Supplementary Fig. 9 and Supplementary Fig. 10 depict the PS I calculated real and imaginary epsilon, respectively. Simulations of light transmission through a bare cavity Supplementary Fig. 11 presents simulations of the electromagnetic field distribution of light transmission through a bare slit at different excitation wavelengths; red (672 nm), green (532 nm) and blue (450 nm). The light distribution reveals only a weak transmission pattern with negligible dependency on the excitation wavelength. Notice that, while excitation of an uncoated slit promotes only weak electromagnetic pattern with comparable signature for all wavelengths, excitation of a microcavity adsorbed with PS I layers ( Fig. 4 ) promotes defined standing wave and a strong SMOL effect. The mode (number of light circles) depends, in this case, on the excitation wavelength and varies between the different excitation bands of the PS I. The simulations highlight the role of the PS I as a nanophotonics filter, which selects the frequencies of photon to interact with the metallic cavity and excite the optical plasmons. The positive sign of the PS I dielectric function facilitates resonant excitation of SP at the cavity and governs the reflection coefficient at the slit metallic interfaces to support the observed standing wave pattern. How to cite this article : Carmeli, I. et al . Spatial modulation of light transmission through a single microcavity by coupling of photosynthetic complex excitations to surface plasmons. Nat. Commun. 6:7334 doi: 10.1038/ncomms8334 (2015).